Molecular memory of prior infections activates the CRISPR/Cas adaptive bacterial immunity system CRISPR/Cas (Clustered Regularly Interspaced Short Palindromic Repeats/CRISPR-associated genes) is a small RNA-based adaptive prokaryotic immunity system that functions by acquisition of short fragments of DNA (mainly from foreign invaders such as viruses and plasmids) and subsequent destruction of DNA with sequences matching acquired fragments. Some mutations in foreign DNA that affect the match prevent CRISPR/Cas defensive function. Here we show that matching sequences that are no longer able to elicit defense, still guide the CRISPR/Cas acquisition machinery to foreign DNA, thus making the spacer acquisition process adaptive and leading to restoration of CRISPR/Cas-mediated protection. We present evidence suggesting that after initial recognition of partially matching foreign DNA, the CRISPR/Cas acquisition machinery moves along the DNA molecule, occasionally selecting fragments to be incorporated into the CRISPR locus. Our results explain how adaptive CRISPR/Cas immunity becomes specifically directed towards foreign DNA, allowing bacteria to efficiently counter individual viral mutants that avoid CRISPR/Cas defense. CRISPRs (clustered regularly interspaced short palindromic repeats) consist of direct repeats separated by spacers of variable sequence [1] , [2] , [3] . Together with associated cas genes [3] , [4] , [5] , CRISPRs provide nucleic acid-based immunity to viruses and plasmids containing sequences matching CRISPR spacers [3] , [6] , [7] , [8] , [9] , [10] . Such sequences are referred to as protospacers [11] . Some mutations in a conserved protospacer-adjacent motif (PAM) [12] prevent CRISPR-mediated immunity (also called 'CRISPR interference'), even when there is a perfect spacer-protospacer match [11] , [13] . Conversely, multiple spacer-protospacer mismatches outside an ~8-bp PAM-proximal protospacer 'seed' region are tolerated without affecting CRISPR immunity, at least in Escherichia coli [13] . In E. coli , a long CRISPR transcript is processed by the CasE endoribonuclease [14] , [15] into a 61-nucleotide CRISPR RNA (crRNA) with 5′-hydroxyl and 2′,3′-cyclic phosphate termini; each crRNA contains a spacer sequence flanked by repeat fragments [14] , [16] . crRNAs are bound by Cascade, a complex composed of CasABCDE proteins [14] , [16] , [17] . Cascade-bound crRNA recognizes DNA containing protospacers matching crRNA spacer [16] , [17] . The presence of PAM increases the strength of interaction 10–50-fold [13] and allows recruitment of Cas3 nuclease required for target DNA cleavage [18] . For CRISPR immunity to occur, a protospacer must first become a spacer during a poorly understood process called 'CRISPR adaptation' [3] , [6] , [7] , [8] , [9] , [10] . E. coli Cas1 and Cas2 proteins are sufficient for spacer acquisition [19] but are dispensable for CRISPR interference [14] . Here we show that in the presence of Cas1, Cas2, Cas3, the Cascade, and crRNA with a sequence matching a phage but no longer able to elicit defense, the CRISPR/Cas acquisition machinery becomes specifically guided to foreign DNA, thus making the spacer acquisition process adaptive and leading to restoration of CRISPR/Cas-mediated protection. We present evidence suggesting that after initial recognition of partially matching foreign DNA, CRISPR/Cas acquisition machinery moves along the DNA molecule, occasionally selecting fragments to be incorporated into the CRISPR locus. This work provides further insight into how the CRISPR/Cas system mediates bacterial immunity. An experimental system to monitor spacer acquisition We studied spacer acquisition in E. coli K12; it contains two CRISPR loci, CRISPR I and CRISPR II (ref. 20 ), and a set of cas genes associated with CRISPR I. When several hundred colonies formed by cells from E. coli culture infected with bacteriophage M13 were screened for spacer acquisition, no CRISPR expansion was detected. As CRISPR interference with M13 infection requires elevated expression of cas genes [13] , which is negatively controlled by global transcription repressor H-NS [15] , [21] , [22] , we switched to a strain with chromosomal cas genes fused to inducible promoters ( Fig. 1a ). Comparisons of total proteins in wild-type E. coli K12 and in induced and uninduced cells with promoter fusions by SDS–PAGE revealed no visible changes, indicating that there was no gross overproduction of Cas proteins in induced cells ( Supplementary Fig. S1 ). Following induction, the engineered cells were infected with M13 at a multiplicity of infection (MOI) of 10, and 300 randomly chosen colonies formed by cells from infected culture were screened for CRISPR expansion. Thirteen clones (~4.3%) acquired new spacers at leader-proximal end of CRISPR II. Four clones acquired spacers from E. coli genome; others acquired phage-derived spacers ( Fig. 1a ; Supplementary Table S1 ). Cells with phage-derived spacers were resistant to M13 only in the presence of inducers. Therefore, the resistance was due to CRISPR interference. Cells with host-derived spacers were phage-resistant both in the presence and in the absence of inducers. Thus, their resistance was CRISPR-unrelated. 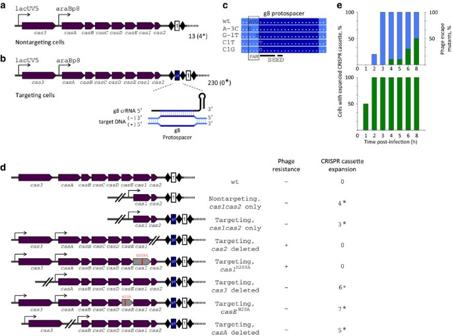Figure 1: CRISPR adaptation ofE. colito M13 requires a preexisting match between CRISPR spacer and phage protospacer. E. coliK12 genomic CRISPR I/caslocus is schematically presented. Individualcasgenes are indicated by purple arrows. Engineered inducible promoters drivingcasgene expression are marked. In nontargeting (a) cells, the CRISPR I consists of 13 spacers (rectangles) and 14 repeats (rhombi). In M13 targeting (b) cells, CRISPR I contains an additional repeat-spacer unit. The new g8 spacer (blue) corresponds to a fragment of M13 gene8and renders cells resistant to wild-type phage infection whencasgene expression is induced. A structure that forms when the g8 crRNA-guided Cascade complex recognizes the double-stranded DNA containing the g8 protospacer is shown below. Numbers to the right of CRISPR/casloci structures show the number of clones (out of 300 tested) that undergone spacer acquisition after infection. Numbers in brackets show the number of clones with host-derived spacers. (c) Progeny phages recovered after nontargeting cell infection have wild-type sequence at and around the g8 protospacer (top). Progeny phage recovered after targeting cell infections contain substitutions at the g8 protospacer PAM or the seed region that lead to escape phenotype. (d) Genetic requirements for CRISPR spacer acquisition. M13 targeting cells carryingcasmutations, shown in column 1, were tested for CRISPR interference ('+' indicates resistance, EOP<10−5; '−' indicates sensitivity, EOP=1, to M13 infection) and ability to acquire new spacers in the course of infection. For each infected culture, 300 randomly chosen colonies were tested for CRISPR expansion and the number of clones that acquired at least one new spacer is provided. Asterisks indicate host-derived spacers. (e) Kinetics of spacer acquisition and escape phage accumulation. The bars show percentages of bacterial clones that underwent CRISPR expansion (green) and percentages of phages harbouring escape mutations at the g8 protospacer or its PAM (blue; top only) at various time points after infection of M13 targeting cells by wild-type (top) and C1T escape (bottom) phages. Representative results of one of three independently conducted experiments are shown. Figure 1: CRISPR adaptation of E. coli to M13 requires a preexisting match between CRISPR spacer and phage protospacer. E. coli K12 genomic CRISPR I/ cas locus is schematically presented. Individual cas genes are indicated by purple arrows. Engineered inducible promoters driving cas gene expression are marked. In nontargeting ( a ) cells, the CRISPR I consists of 13 spacers (rectangles) and 14 repeats (rhombi). In M13 targeting ( b ) cells, CRISPR I contains an additional repeat-spacer unit. The new g8 spacer (blue) corresponds to a fragment of M13 gene 8 and renders cells resistant to wild-type phage infection when cas gene expression is induced. A structure that forms when the g8 crRNA-guided Cascade complex recognizes the double-stranded DNA containing the g8 protospacer is shown below. Numbers to the right of CRISPR/ cas loci structures show the number of clones (out of 300 tested) that undergone spacer acquisition after infection. Numbers in brackets show the number of clones with host-derived spacers. ( c ) Progeny phages recovered after nontargeting cell infection have wild-type sequence at and around the g8 protospacer (top). Progeny phage recovered after targeting cell infections contain substitutions at the g8 protospacer PAM or the seed region that lead to escape phenotype. ( d ) Genetic requirements for CRISPR spacer acquisition. M13 targeting cells carrying cas mutations, shown in column 1, were tested for CRISPR interference ('+' indicates resistance, EOP<10 −5 ; '−' indicates sensitivity, EOP=1, to M13 infection) and ability to acquire new spacers in the course of infection. For each infected culture, 300 randomly chosen colonies were tested for CRISPR expansion and the number of clones that acquired at least one new spacer is provided. Asterisks indicate host-derived spacers. ( e ) Kinetics of spacer acquisition and escape phage accumulation. The bars show percentages of bacterial clones that underwent CRISPR expansion (green) and percentages of phages harbouring escape mutations at the g8 protospacer or its PAM (blue; top only) at various time points after infection of M13 targeting cells by wild-type (top) and C1T escape (bottom) phages. Representative results of one of three independently conducted experiments are shown. Full size image Phage protospacers from which spacers were derived had a functional AAG PAM [18] ( Supplementary Table S1 ). Protospacers from bacterial genome were associated with AAT, TTA, ACT, and ACG sequences that do not match the PAM consensus [12] . M13 mutants with ACG or AAT introduced instead of a functional PAM exhibit an 'escape' phenotype [13] , [18] : they infect 'targeting' cells containing an M13-derived spacer with an EOP (efficiency of plaquing, defined as the ratio of number of phage plaques formed on targeting cell lawns to the number of plaques formed on wild-type cell lawns) of one [18] . Wild-type phage infects targeting cells with an EOP<10 −5 . No spacer acquisition was detected in uninfected culture, suggesting that increased Cas levels and phage infection are jointly required for spacer acquisition. However, the process is inefficient under the conditions tested and not selective for phage DNA. The actual number of host-derived spacer acquisition events must be higher than detected, because cells that acquire spacers from protospacers with functional PAM must mount a self-immunity response and die [23] . Phage-matching spacers stimulate M13-derived spacers acquisition Seven out of nine clones that acquired phage-derived spacers had multiple spacers ( Supplementary Table S1 ) suggesting that first spacer insertion stimulates subsequent acquisitions. Therefore, spacer acquisition experiment was repeated with M13-resistant targeting cells containing engineered CRISPR I with a spacer matching a fragment of M13 gene 8 (the 'g8' spacer [13] ; Fig. 1b ). Induced targeting cells were infected at MOI=10 with wild-type phage, and 300 colonies formed by cells from infected cultures were analysed for CRISPR expansion. CRISPR expansion was detected in 77% (230) of clones ( Fig. 1b ), with 17% of expansions occurring in CRISPR I and the rest in CRISPR II. The apparent preference for spacer acquisition in CRISPR II could be caused by the differences in the leader sequence in front of the first repeat [19] , or caused by higher level of transcription of CRISPR II (ref. 15 ); this matter requires further investigation. The same high frequency of spacer acquisition was observed when g8 spacer was inserted in CRISPR II or when spacers matching protospacers in M13 gene 1 or 2 were inserted in CRISPR I. All spacers were phage-derived with many clones acquiring multiple spacers ( Supplementary Table S2 ). We conclude that spacer acquisition is strongly stimulated and becomes adaptive, that is, targeted to phage DNA, when CRISPR spacer matches phage protospacer. We refer to this phenomenon as 'priming'. More than 97% (176 of 181) of phage protospacers that served as a source of new spacers were associated with an AAG PAM. Phages that form plaques on induced targeting cell lawns acquire 'escape' mutations that inactivate g8 PAM or protospacer ( Fig. 1c ). Cells containing new phage-derived spacers were resistant to both the wild-type and escape phages carrying substitutions in g8 protospacer or PAM. Phages that infected cells with newly acquired spacers invariably contained double mutations in both g8 protospacer/PAM and protospacer/PAM corresponding to new spacer ( Supplementary Fig. S2 ). Thus, new phage-derived spacers are capable of interference, as expected. Genetic requirements for primed spacer acquisition Only low-level acquisition of host-derived spacers was observed during infection of targeting or non-targeting cells expressing just cas1 and cas2 ( Fig. 1d , Supplementary Tables S3 and S4 ). Cells lacking cas2 , or producing Cas1 point mutant lacking nucleolytic activity [24] , did not acquire spacers ( Fig. 1d ). Low-level incorporation of host-derived spacers was also observed in targeting cells lacking cas3 ( Fig. 1d ; Supplementary Table S5 ); with mutation inactivating the CasE endonuclease ( Fig. 1d ; Supplementary Table S6 ), or lacking casA ( Fig. 1d ; Supplementary Table S7 ). Thus, primed adaptive acquisition of phage-derived spacers requires a crRNA-matching phage protospacer, Cascade, Cas1, Cas2, and Cas3. Primed spacer acquisition is driven by phages escape mutants Individual phages from infected targeting and nontargeting cultures were isolated, and DNA sequences at and around the g8 protospacer determined. Phages from nontargeting cells infection had a wild-type sequence. Phages from targeting cells infection contained escape mutations in g8 protospacer or PAM ( Fig. 1c ). Thus, acquisition of phage-derived spacers may be initiated by rare escape phages present in wild-type phage sample. Indeed, no spacer acquisition was detected in cultures infected with wild-type phage at MOI=10 −3 , when the number of phages was so low that no spontaneous escape mutants were expected. Conversely, robust spacer acquisition was observed when targeting cells were infected at low MOI of 10 −3 with escape phage carrying a C1T substitution in g8 protospacer seed region. During MOI=10 escape phage infection, spacer acquisition was detected as early as one hour post-infection ( Fig. 1e ). During wild-type infection at MOI of 10, a significant fraction of clones with new spacers was detected only six hours post-infection and their appearance was preceded by accumulation of escape phages ( Fig. 1e ). The same result was obtained with escape phage carrying a g8 PAM G-1T mutation. In contrast, in the course of infection with escape phage carrying a double mutation G-1T C1T only low-level acquisition of host-derived spacers was observed ( Supplementary Fig. S3 ), indicating that priming was prevented. The last PAM nucleotide is inserted along with protospacer When a new spacer is inserted, an extra repeat is also generated from promoter-proximal, first, repeat [19] . The first CRISPR II repeat has a CCG sequence at the 'PAM-side' of the spacer. Extra repeats in cells that acquired new spacers contained, in addition to exact copies ending with CCG, occasional versions ending with CCA, CCT and CCC. Swarts et al . [25] analysed E. coli CRISPR repeat polymorphisms and suggested that they may be determined by PAM base closest to protospacer (position -1). Analysis of an extensive collection of spacer polymorphisms and corresponding M13 protospacers further strengthens the hypothesis of Swarts et al . ( Fig. 2a ). An experimental proof was also obtained by generating targeting strains with mutated first CRISPR II repeat, performing an acquisition experiment, and determining extra repeat sequences (all new spacers were derived from protospacers with AAG PAM). A substitution of G to T at repeat position -1 (G-1T) was not passed on to new repeats, which contained a G at the -1 position, while an A-4G substitution was inherited by all new repeats ( Fig. 2b ). When engineered repeat carried C-2A and G-1T double substitution, new repeats had an A at position -2 but a G at position -1 ( Fig. 2b ). Thus, base pair at repeat position -1 is determined by a base pair at the corresponding PAM position. In other words, the entire protospacer and the last residue of PAM are inserted in CRISPR cassette ( Fig. 2c ). 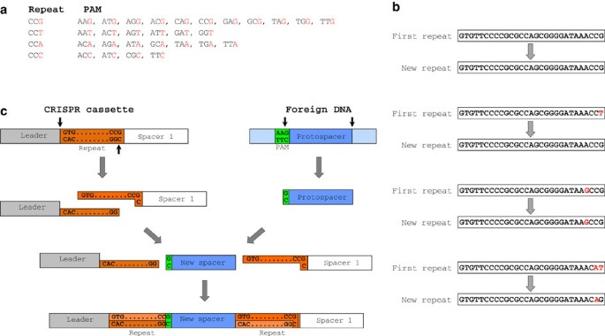Figure 2: Repeat polymorphisms are determined by the last base of PAM of protospacers from which the spacers are acquired. (a) The last three bases of new repeat copies and PAMs of protospacers from which associated spacers are derived are shown. (b) The sequences of new repeats copies generated after acquisition of spacers from M13 protospacers with AAG PAM are shown. Strains used in spacer acquisition experiments contained either a wild-type CRISPR (top) or a CRISPR array with engineered substitutions in the first repeat (highlighted in red). (c) A mechanism of spacer insertion (ref.25) consistent with data presented in panelsaandb. Figure 2: Repeat polymorphisms are determined by the last base of PAM of protospacers from which the spacers are acquired. ( a ) The last three bases of new repeat copies and PAMs of protospacers from which associated spacers are derived are shown. ( b ) The sequences of new repeats copies generated after acquisition of spacers from M13 protospacers with AAG PAM are shown. Strains used in spacer acquisition experiments contained either a wild-type CRISPR (top) or a CRISPR array with engineered substitutions in the first repeat (highlighted in red). ( c ) A mechanism of spacer insertion (ref. 25 ) consistent with data presented in panels a and b . Full size image Analysis of spacer acquisition strand bias Genomic locations of M13 protospacers from which spacers were acquired during targeting cells infection are shown in Fig. 3b . 88% (160 out of 181) spacers originated from non-transcribed genome strand. No such bias was observed for protospacers from which spacers were acquired during nontargeting infection (10 out of 29, Fig. 3a ). The preferred orientation (with respect to PAM) of protospacers from which spacers are acquired during targeting cell infection matches the orientation of the priming g8 protospacer. A similar protospacer distribution was observed with cells expressing crRNAs targeting protospacers located in M13 gene 1 or 2 ( Supplementary Fig. S4 ). To determine the role of priming protospacer in spacer selection, two plasmids carrying the ampicillin resistance bla gene and an M13 fragment with g8 protospacer cloned in opposite orientations were transformed into targeting cells expressing cas genes. Ampicillin-resistant transformants were grown without ampicillin to allow plasmid loss, and resulting ampicillin-sensitive colonies were monitored for spacer acquisition. 23% (99 out of 430) of targeting cell clones contained expanded CRISPR II. The number was increased to 85% (81 out of 95 clones) when a plasmid with C1T escape mutation in g8 protospacer was used, confirming that escape mutations stimulate primed spacer acquisition. All new spacers were plasmid-derived and corresponding protospacers were unequally distributed, with strand bias matching the orientation of g8 protospacer in each plasmid ( Fig. 4 ; Supplementary Tables S8 and S9 ). 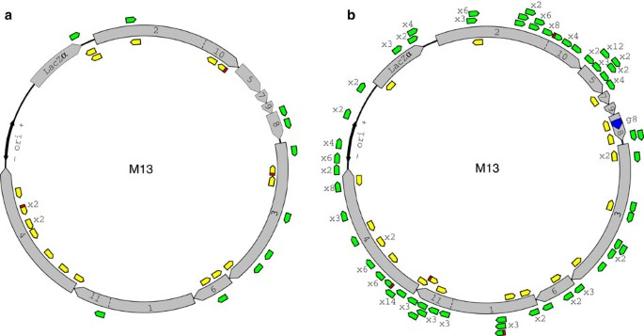Figure 3: Distribution of acquired M13 spacers in the M13 genome. The double-stranded 7,249 bp circular replicative form of the M13mp18 genome is shown with individual genes indicated. Protospacers corresponding to newly acquired phage-derived spacers, during M13 nontargeting (a) and targeting (b) cell infections, are indicated by green (protospacers located in the coding strand of the M13 genome) and yellow (protospacers located in the noncoding strand of the M13 genome) arrows. The arrows are pointing away from the PAM sequence. Protospacers in green or yellow only contain an AAG version of PAM. Protospacers marked in red contain other PAM sequences. Numbers indicate the number of times identical spacers have been observed. In panelb, the g8 protospacer is indicated by a blue arrow. Figure 3: Distribution of acquired M13 spacers in the M13 genome. The double-stranded 7,249 bp circular replicative form of the M13mp18 genome is shown with individual genes indicated. Protospacers corresponding to newly acquired phage-derived spacers, during M13 nontargeting ( a ) and targeting ( b ) cell infections, are indicated by green (protospacers located in the coding strand of the M13 genome) and yellow (protospacers located in the noncoding strand of the M13 genome) arrows. The arrows are pointing away from the PAM sequence. Protospacers in green or yellow only contain an AAG version of PAM. Protospacers marked in red contain other PAM sequences. Numbers indicate the number of times identical spacers have been observed. In panel b , the g8 protospacer is indicated by a blue arrow. 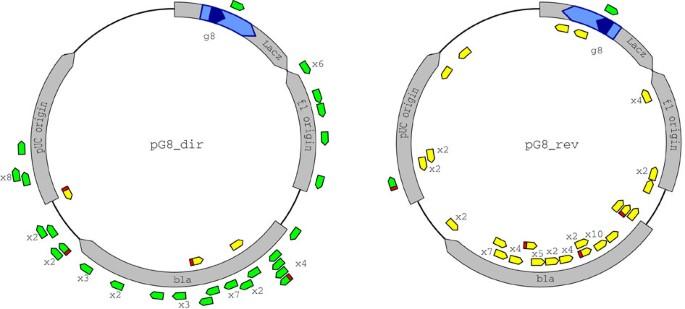Figure 4: The priming spacer orientation influences the choice of new spacers. Two plasmids with opposing orientations of M13 fragment (light blue) containing the g8 protospacer (dark blue arrow) are schematically shown. Protospacers corresponding to spacers acquired by cells that lost each plasmid are shown as green (protospacers located in the coding strand of ampicillin-resistance genebla) and yellow (protospacers located in the noncoding strand ofbla) arrows. Protospacers marked in red contain other than AAG PAM sequences. Numbers indicate the number of times identical spacers have been observed. Full size image Figure 4: The priming spacer orientation influences the choice of new spacers. Two plasmids with opposing orientations of M13 fragment (light blue) containing the g8 protospacer (dark blue arrow) are schematically shown. Protospacers corresponding to spacers acquired by cells that lost each plasmid are shown as green (protospacers located in the coding strand of ampicillin-resistance gene bla ) and yellow (protospacers located in the noncoding strand of bla ) arrows. Protospacers marked in red contain other than AAG PAM sequences. Numbers indicate the number of times identical spacers have been observed. Full size image Here we showed that in E. coli , efficient CRISPR adaptation requires spacers matching the foreign genome. At first glance, this seems to be counterintuitive, for the presence of such spacers means that the host is already resistant to invading genetic element. However, point substitutions in PAM or protospacer, which abolish CRISPR interference and strongly decrease the affinity of the Cascade-crRNA complex to target DNA [13] , actually stimulate spacer acquisition. Therefore, the weakened interaction of Cascade-crRNA complex with protospacers allows bacteria to 'recall' prior infections and triggers robust acquisition of new phage-derived spacers, provided that enough Cas1 and Cas2 are present. This is clearly beneficial to the host as it allows it to 'adapt' and become resistant to escape phages that avoid interference by older spacers. The same process can also induce spacer acquisition when the priming spacer provides only partial protection from phage infection, leading to increased immunity. Accumulation of additional mutations in PAM or protospacer abolishes the molecular memory of prior encounters by further decreasing or completely abolishing target recognition. This phenomenon is likely responsible for suppression of self-priming on CRISPR, because crRNA-Cascade complex does not interact with targets containing repeat sequences [17] , [26] . In the absence of priming, both host- and phage-derived spacers are acquired with low efficiency in a Cascade- and Cas3-independent but Cas1/Cas2-dependent process (schematically illustrated in Fig. 5a ). Acquisition of phage-derived spacers allows bacteria to mount CRISPR interference; only phages with escape mutations can infect such cells ( Fig. 5b ). However, during escape phage infection, the cells can mount a highly efficient Cascade-, Cas3-, and Cas1/Cas2-dependent adaptive acquisition of additional phage-derived spacers through priming ( Fig. 5c ). As a result, many bacteria acquire multiple resistance determinants (that is, spacers) and become totally resistant to the phage. 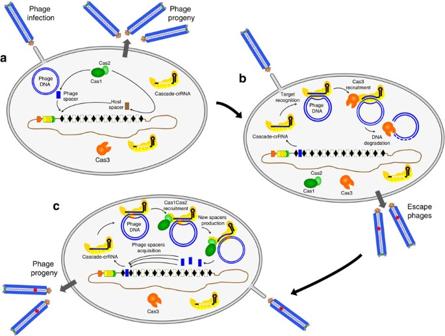Figure 5: A summary of CRISPR spacer acquisition in M13-infectedE. coli. (a) During infection of 'naïve' cells without M13-targeting spacers low-level Cas1/Cas2-dependent, Cascade-, Cas3-independent acquisition of spacers takes place. Both host and phage-derived spacers are acquired. (b) Cells that acquire phage-derived spacers become resistant to wild-type phage through CRISPR interference, however, are subject to productive infection by escape phages. (c) When a cell harbouring a phage-derived spacer is infected by an escape phage, adaptive acquisition of multiple new phage-derived spacers is triggered through priming interaction of Cascade complexed with crRNA containing phage-derived spacer with a protospacer harbouring an escape mutation, leading to cells that are able to block infection with escape phages. The process requires Cas1, Cas2, and Cas3. Figure 5: A summary of CRISPR spacer acquisition in M13-infected E. coli . ( a ) During infection of 'naïve' cells without M13-targeting spacers low-level Cas1/Cas2-dependent, Cascade-, Cas3-independent acquisition of spacers takes place. Both host and phage-derived spacers are acquired. ( b ) Cells that acquire phage-derived spacers become resistant to wild-type phage through CRISPR interference, however, are subject to productive infection by escape phages. ( c ) When a cell harbouring a phage-derived spacer is infected by an escape phage, adaptive acquisition of multiple new phage-derived spacers is triggered through priming interaction of Cascade complexed with crRNA containing phage-derived spacer with a protospacer harbouring an escape mutation, leading to cells that are able to block infection with escape phages. The process requires Cas1, Cas2, and Cas3. Full size image The DNA strand from which new spacers are selected is largely determined by the priming protospacer orientation. We propose that after initial low-affinity priming interaction of the Cascade-crRNA complex with a protospacer harbouring an escape mutation, the complex slides along the target DNA until a PAM sequence is reached, and a process that leads to new spacer insertion commences. Molecular details of this process remain to be elucidated, but it is clear that the last base of PAM and the protospacer are jointly inserted into recipient CRISPR. The distribution of protospacers in plasmid and M13 genomes with respect to priming protospacer locations suggests that efficiency of PAM recognition during selection of protospacers for acquisition is rather low, because multiple copies of functional PAM sequences seem to be bypassed en route to most successful spacer acquisition events. During 'primed' CRISPR adaptation, a host that acquired a spacer from a particular phage should acquire additional spacers from this or very similar phages with higher frequency. Indeed, despite the general paucity of E. coli spacers matching known phages, in the exceptional case of E. coli strains E24377A and SE11 34 spacers targeting a single phage have been revealed [20] . Bioinformatic analysis of metagenomic data suggests that facilitated spacer acquisition also operates during CRISPR-mediated co-evolution of archaea and their viruses [27] . Thus, facilitated adaptive spacer acquisition directed by recognition of foreign DNA that is no longer subject to CRISPR interference might be an evolutionary conserved feature of all CRISPR systems. Bacterial strains and plasmids E. coli strains used are listed in Supplementary Table S10 . Strains with site-specific mutations were engineered using a simple two-step mutagenesis procedure based on the use of the Red recombinase [28] . Plasmids pWUR397 (expressing cas 3), pWUR399 (co-expressing casABCDE12 ), pWUR477 (expressing nontargeting CRISPR), and its targeting derivative containing g8 spacer have been described previously [13] , [14] . pG8_dir or pG8_rev plasmids carry a 209-bp M13 fragment containing the g8 protospacer (genome positions 1311–1519) cloned into the Eco RV site of the pT7Blue blunt-end vector (Novagen). Spacer acquisition experiments To monitor spacer acquisition during phage infection, overnight cultures of appropriate cells were diluted 100-fold into fresh LB medium containing 1 mM isopropyl-β- D -thiogalactoside (IPTG) and arabinose and grown at 37 °C, until OD 600 reached 0.4–0.5. Cultures were combined with phage lysates to reach an appropriate MOI and, after a 5-min incubation at 37 °C without agitation, and 15 min at 37 °C with agitation cultures, diluted tenfold into fresh medium containing IPTG and arabinose. Infections continued at 37 °C for various times. Culture aliquots were spread on LB agar plates containing IPTG and arabinose. Plates were incubated at 37 °C until individual colonies appeared. To monitor spacer acquisition in plasmid-transformed cells, E. coli BW39908 derivatives carrying pWUR397, pWUR399 and pWUR477 or their targeting derivative were transformed with pG8_dir or pG8_rev. Individual ampicillin-resistant colonies were grown overnight in liquid LB with 25 μg ml −1 Str, 25 μg ml −1 Kan, 34 μg ml −1 Cam. Culture aliquots were spread on LB agar plates supplemented with 25 μg ml −1 Str, 25 μg ml −1 Kan, 34 μg ml −1 Cam and individual colonies tested for ability to grow in the presence of 100 μg ml −1 Amp. Ampicillin-sensitive colonies were screened for CRISPR expansion. CRISPR expansion was monitored by PCR using appropriate primer pairs amplifying promoter–proximal ends of CRISPR I and CRISPR II (ref. 20 ). For CRISPR I amplification, primers Ec_LDR_F (5′-AAGGTTGGTGGGTTGTTTTTATGG-3′) and Ec_I_sp2 (5′-CGGCATCACCTTTGGCTTCGGCTG-3′) were used. For CRISPR II amplification, primers Ec_II F (5′-AACATAATGGATGTGTTGTTTGTG-3′) and Ec_II R (5′-GAAATGCTGGTGAGCGTTAATG-3′) were used. How to cite this article: Datsenko, K. A. et al . Molecular memory of prior infections activates the CRISPR/Cas adaptive bacterial immunity system. Nat. Commun. 3:945 doi: 10.1038/ncomms1937 (2012).